Large influence of atmospheric vapor pressure deficit on ecosystem production efficiency 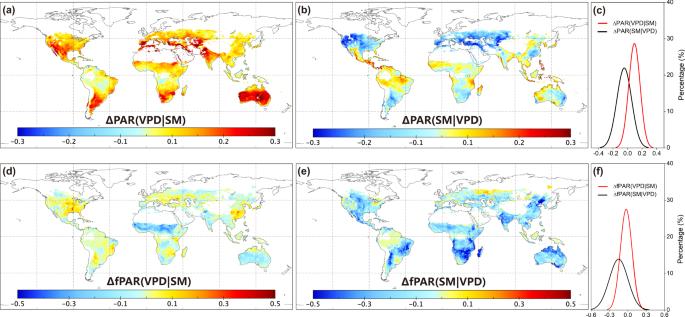Fig. 1: Effects of soil moisture (SM) and vapor pressure deficit (VPD) on photosynthetically active radiation (PAR) and fraction of photosynthetically active radiation absorbed by plants (fPAR) globally. a,bIndicate the spatial distribution of the changes in PAR caused by high VPD (ΔPAR(VPD|SM)) and low soil moisture (SM) (ΔPAR(SM|VPD)), andcshows the probability density function of ΔPAR.d–fIndicate the corresponding changes of fPAR. For better comparability in space, the PAR and fPAR data time series were normalized by the average exceeding 90th percentile per pixel. The units refer to the fractions relative to average PAR and fPAR exceeding the 90th percentile in each grid cell. Regions with sparse vegetation and regions without valid data are masked in white. This analysis followed the method of Liu et al. [1] to quantify the respective impacts of SM and VPD on ecosystem production. To isolate the coincident impacts of PAR and fPAR on ecosystem production, we use fluorescence quantum yield (SIF yield ) and light use efficiency (LUE) instead of SIF used by Liu et al. [1] , to better indicate the capacity of vegetation production [3] , [12] : 
    SIF_yield=SIF/PAR × fPAR
 (1) 
    LUE=GPP/PAR × fPAR
 (2) where PAR and fPAR indicate photosynthetically active radiation and fraction of photosynthetically active radiation respectively. LUE was calculated at both site-scale using EC measurements from 40 sites and global scale using global model data (i.e., FLUXCOM). The same data selection criterion of Liu et al. [1] is followed at global scale, i.e., only SM or VPD bins where >10 data points are available. At site-scale, the threshold for LUE is set to 5 due to limited data availability. 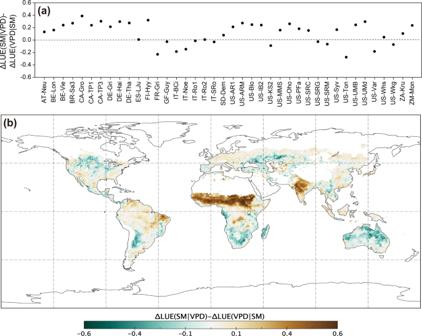Fig. 2: The comparison on impacts of soil moisture (SM) and vapor pressure deficit (VPD) on ecosystem light use efficiency (LUE) based on measurements of eddy covariance sites and global model data. aDifferences between ΔLUE(SM|VPD) and ΔLUE(VPD|SM) at 40 eddy covariance sites.bDifferences between ΔLUE(SM|VPD) and ΔLUE(VPD|SM) based on FLUXCOM dataset. The positive values indicate larger impacts of VPD relative to SM ina,b. Note, where ΔLUE(SM|VPD)>0, the difference equals to ΔLUE(VPD|SM) ina,b; where ΔLUE(VPD|SM)>0, the difference is ΔLUE(SM|VPD); and where both are positive, the difference is not shown. For better comparability in space, the LUE data time series was normalized by the average LUE exceeding 90th percentile. The units refer to the fractions relative to average LUE exceeding the 90th percentile for each eddy covariance site and each grid cell. All datasets are listed in Supplementary Table 2 .